Unique fingering instabilities and soliton-like wave propagation in thin acoustowetting films There has long been substantial interest in the wetting of thin liquid films given the rich diversity of phenomena associated with non-linear spreading dynamics, including self-similar fractal assembly, finger patterning and self-organisation [1] , [2] , [3] , [4] , [5] , [6] . In addition to their prevalence in nature, their relevance to micro- and nano-scale processes have led to closer scrutiny of such phenomena in the context of microfluidic research [7] , [8] , [9] , [10] . Similarly, the interaction of sound waves and vibrations with fluids has an equally rich history dating back to Faraday’s [11] observation of capillary waves on vertically vibrated substrates and Rayleigh’s [12] description of acoustic streaming in air-filled resonant tubes. It has, however, only been in the last decade that renewed interest has emerged in the subject, particularly surrounding flows arising from nanometer amplitude high-frequency (MHz order) substrate vibration in the form of surface acoustic waves (SAWs) [13] , not only because of their tremendous potential for driving a variety of microfluidic operations such as drop transport [14] , fluid mixing [15] and particle/cell alignment [16] , but also because of the recent discovery of associated phenomena such as dynamic colloidal patterning [17] and interfacial jetting [18] . Here we report on a novel collection of dynamic spreading and flow-instability phenomena that arise when a sessile fluid drop is subjected to the SAW. Quite non-intuitively, a thin film is observed to be drawn out from the drop in a direction that opposes that of the SAW propagation due to the dominant Rayleigh streaming in the film. Fresnel diffraction of the acoustic wave as a consequence of the finite aperture of the electrodes used to generate the SAW, however, leads to transverse variations in the speed at which the film front advances, in turn driving a front instability reminiscent of, but distinct from, viscous and granular fingering instabilities [19] , [20] , [21] , [22] , [23] . Finally, rather unique ‘soliton-like’ wave train pulses were observed to grow above these fingers; these are subsequently transported away along the propagation direction of the SAW under the influence of long-range Eckart streaming that dominates when the wave pulses grow beyond a critical height commensurate with the SAW wavelength. In addition to deriving a dynamic spreading model from which we find good agreement with our experimental observations, we show the competing influence of Rayleigh and Eckart streaming responsible for the observed flow reversal at different length scales. 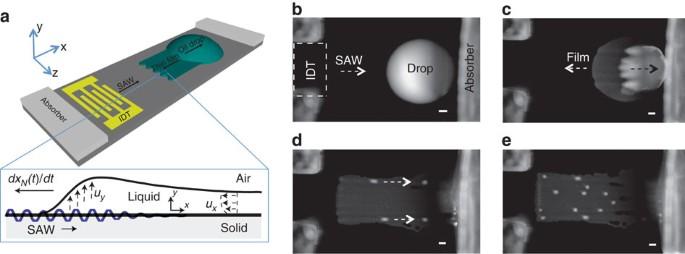Figure 1:Experimental setup and acoustowetting phenomena. (a) Schematic illustration of the experimental setup depicting the emergence of a thin film from a sessile oil drop under the influence of a propagating SAW. The inset is a side view sketch of the film’s leading edge, advancing with velocitydxN(t)/dt;xN(t) is the position of the film front as it advances with timetand the characteristic flow field in the film is denoted by (ux,uy). The panel on the right depicts a sequence of top-view images of the drop, fluorescently labelled to aid visualisation, (b) in its initial state, which (c) on subsequent excitation with the SAW, is displaced along the SAW propagation direction while forming a 20-μm thick film that advances in the opposite direction. (d) This film later suffers from a transient instability that gives rise to the formation of fingering patterns. ‘Soliton-like’ wave pulses subsequently appear above the fingers and translate away in the SAW propagation direction, first along the side edges of the film, and then (e) across the entire film. The scale bars denote lengths of ≈1 mm, and the bright corners at the left side of the images are the electrical connections to the IDT. Acoustowetting and associated phenomena Figure 1 illustrates this curious triad of film spreading, fingering instabilities and ‘soliton-like’ wave pulses collectively triggered from a sessile drop by the SAW; a description of the experimental setup ( Fig. 1a ) is provided in the Methods section, whereas a video capturing the phenomena is included in the Supplementary Information . Analogous to spontaneous electrowetting [24] , [25] , [26] , acoustowetting films are, however, not a result of a direct stress (or stress gradient) on the interface unlike their electrohydrodynamic counterpart, but emanate as a consequence of the drift flow arising from Rayleigh streaming [12] . Although both advancing and trailing thin films under SAW excitation have previously been observed [27] , [28] , there has yet to be an explanation of how they appear and why they spread, quite unusually, in a direction opposing that of the SAW propagation. Parenthetically, we note that atomisation of the liquid at the meniscus front due to the SAW, deposition of the atomised droplets ahead of the front and their subsequent coalescence with the contact line front has previously been proposed as a collective mechanism to explain the counterpropagating advancing front in a confined microchannel, although little evidence has been provided in support of this hypothesis [29] . Moreover, not only is the speed of the advancing front and its dependency on the various system parameters markedly different in the present case, we also did not observed any atomisation, mainly because of the low SAW power employed, which is insufficient to drive interfacial destabilisation of the viscous oils used. Figure 1: Experimental setup and acoustowetting phenomena. ( a ) Schematic illustration of the experimental setup depicting the emergence of a thin film from a sessile oil drop under the influence of a propagating SAW. The inset is a side view sketch of the film’s leading edge, advancing with velocity dx N ( t )/ dt ; x N ( t ) is the position of the film front as it advances with time t and the characteristic flow field in the film is denoted by ( u x , u y ). The panel on the right depicts a sequence of top-view images of the drop, fluorescently labelled to aid visualisation, ( b ) in its initial state, which ( c ) on subsequent excitation with the SAW, is displaced along the SAW propagation direction while forming a 20-μm thick film that advances in the opposite direction. ( d ) This film later suffers from a transient instability that gives rise to the formation of fingering patterns. ‘Soliton-like’ wave pulses subsequently appear above the fingers and translate away in the SAW propagation direction, first along the side edges of the film, and then ( e ) across the entire film. The scale bars denote lengths of ≈1 mm, and the bright corners at the left side of the images are the electrical connections to the IDT. Full size image A more likely explanation for the counterpropagating film front lies in the various streaming mechanisms that can arise in a liquid body that is acoustically excited. On the one hand, the parent drop of thickness L E ≈1 mm allows the attenuation of SAW-induced sound waves in the bulk of the fluid over length scales many times the sound wavelength λ l (≈77 and 46 μm at the SAW frequencies employed, f =19.5 and 32.7 MHz, respectively), that is, , therefore supporting the usually dominant Eckart streaming [30] . Consequently, the net fluid motion and hence the displacement of the drop is along the SAW propagation direction ( Fig. 1c ). On the other hand, the thickness of the thin film H ≈20 μm < λ l is insufficient to support the formation of bulk sound waves within, therefore suppressing Eckart streaming. In this case, Rayleigh streaming then dominates. We show below that a spatially decaying vertical velocity arises at the free surface due to the Rayleigh streaming, which, together with mass conservation in the film, drives the film to spread in a direction opposing that of the SAW propagation ( Fig. 1c ). Film spreading A more stringent condition for the formation of a film from a sessile drop can then be envisaged, which depends on the wettability of the fluid: only drops with sufficiently small contact angles θ ≈ H / L (for example, θ≈ 10°–25° for silicone oil) such that H < λ l permit Rayleigh streaming to dominate over a confined region on the order of λ l near the contact line, drawing out a thin front-running acoustowetting film. In contrast, translation of the entire sessile drop, without film spreading, is observed when fluids with large contact angles such as water ( θ ≈60°) or glycerol ( θ ≈70°) are used because no such Rayleigh streaming-dominant regions can form. To verify our hypothesis, we rendered the substrate more hydrophillic to water and glycerol through plasma etching of the substrate in air and found that the onset of film formation only occurs when the contact angle of these fluids is decreased below 30°. In addition, rendering the substrate more oleophobic to silicone oil by patterning its surface with a 100-nm thick Teflon AF layer suppresses the formation of the thin film. We provide a more rigorous verification of the dominant role of Rayleigh streaming in the film-spreading process by deriving an expression for the temporal displacement of the advancing contact line. Given H < λ l , it is reasonable to neglect the contribution to the flow due to Eckart streaming [13] and solve the equations governing mass and momentum conservation in a confined region in the vicinity of the three-phase contact line at the advancing film front (the derivation is provided in the Supplementary Information ); the film is bounded between a periodic displacement boundary condition imposed by the Rayleigh SAW propagation along the solid substrate and a stress-free boundary condition imposed by the free surface. Briefly, the leading-order steady component of the Rayleigh streaming at the free surface imposes a vertical upward velocity at the free surface that decays away from the leading edge of the film as the SAW attenuates. Together with a kinematic boundary condition at the free surface that imposes mass conservation in the spatiotemporally evolving film, we observe the film to spread with a constant velocity in a direction opposite to that of the SAW propagation. When scaled with the SAW wavelength λ SAW , the position of the advancing film front x N as a function of time t reads where is a characteristic spreading time scale, in which is the Mach number in the solid and is the viscous penetration length. ρ and μ are the fluid density and viscosity, respectively, U is the substrate (SAW) displacement velocity amplitude, c SAW is the propagation speed of the SAW of frequency f and φ=3 π /2 is the phase difference between its longitudinal and transverse components, which have roughly the same amplitude. We note that the streaming Reynolds number [13] is small, indicating that the spreading of the film is driven by a weak convective mechanism—Stokes drift—invoked by the viscous-dominant Rayleigh streaming in the film. Not only is the linear relationship in equation (1) in qualitative agreement with the experimental observations presented in Fig. 2a , but there is also very good quantitative agreement between our theoretical prediction and the experimental results (see Fig. 2a , inset), remarkably in the absence of any empirical fitting parameters. This inspires confidence in the proposed Rayleigh streaming theory as the underlying film-spreading mechanism. Further comparison between the theoretically predicted and experimentally measured film velocities over a range of SAW amplitudes and frequencies, and fluid viscosities is given in Fig. 2b . 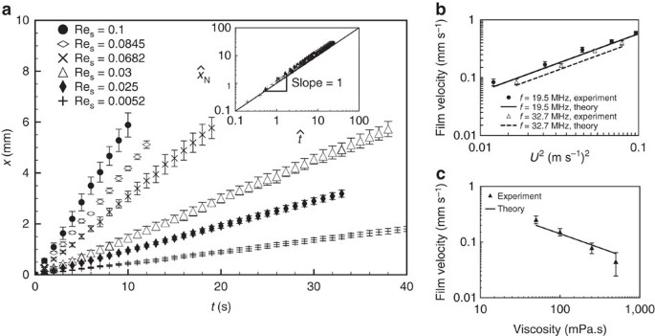Figure 2:Dynamics of the spreading film. (a) Displacement of the advancing film frontxNwith timetas a function of the substrate (SAW) displacement velocityU, fluid viscosityμand frequencyf, parameterised by the streaming Reynolds number Res. The same experimental data is replotted in dimensionless form in the inset by normalisingxNandtwith the scaling apparent in equation (1), that is,and, whereλSAWis the SAW wavelength andtcis the characteristic spreading time scale; the collapse of the data with the universal spreading law derived indicates the excellent agreement between the theoretical prediction and experimental observations. Legend: +:U=0.16 m s−1,μ=500 mPa.s,f=19.5 MHz (Res=0.0052,β−1=1.14 × 10−6m);:U=0.13 m s−1,μ=50 mPa.s,f=32.7 MHz (Res=0.025,β−1=2.78 × 10−7m); Δ:U=0.185 m s−1,μ=100 mPa.s,f=19.5 MHz (Res=0.03,β−1=5.1 × 10−7m); × :U=0.21 m s−1,μ=50 mPa.s,f=19.5 MHz (Res=0.0682,β−1=3.6 × 10−7m);:U=0.26 m s−1,μ=50 mPa.s,f=19.5 MHz (Res=0.0845,β−1=3.6 × 10−7m);:U=0.31 m s−1,μ=50 mPa.s,f=19.5 MHz (Res=0.1,β−1=3.6 × 10−7m).β−1is the viscous penetration length. Two distinct devices were used to generate the two SAW frequencies reported in the data set. The subfigures on the right portray the variation in the velocity of the advancing film front with (b) the substrate (SAW) displacement velocity amplitudeUand (c) the fluid viscosity, showing the comparison between the experimental data and the theoretical prediction given by equation (1). In the former the fluid viscosity is held constant at 100 mPa.s, and in the latterU=0.185 m s−1. The SAW frequency is fixed at 19.5 MHz in the latter case. In all cases, error bars denote the s.e. forn=3 runs for each data set. Figure 2: Dynamics of the spreading film. ( a ) Displacement of the advancing film front x N with time t as a function of the substrate (SAW) displacement velocity U , fluid viscosity μ and frequency f , parameterised by the streaming Reynolds number Re s . The same experimental data is replotted in dimensionless form in the inset by normalising x N and t with the scaling apparent in equation (1), that is, and , where λ SAW is the SAW wavelength and t c is the characteristic spreading time scale; the collapse of the data with the universal spreading law derived indicates the excellent agreement between the theoretical prediction and experimental observations. Legend: +: U =0.16 m s −1 , μ =500 mPa.s, f =19.5 MHz (Re s =0.0052, β −1 =1.14 × 10 −6 m); : U =0.13 m s −1 , μ =50 mPa.s, f =32.7 MHz (Re s =0.025, β −1 =2.78 × 10 −7 m); Δ: U =0.185 m s −1 , μ =100 mPa.s, f =19.5 MHz (Re s =0.03, β −1 =5.1 × 10 −7 m); × : U =0.21 m s −1 , μ =50 mPa.s, f =19.5 MHz (Re s =0.0682, β −1 =3.6 × 10 −7 m); : U =0.26 m s −1 , μ =50 mPa.s, f =19.5 MHz (Re s =0.0845, β −1 =3.6 × 10 −7 m); : U =0.31 m s −1 , μ =50 mPa.s, f =19.5 MHz (Re s =0.1, β −1 =3.6 × 10 −7 m). β −1 is the viscous penetration length. Two distinct devices were used to generate the two SAW frequencies reported in the data set. The subfigures on the right portray the variation in the velocity of the advancing film front with ( b ) the substrate (SAW) displacement velocity amplitude U and ( c ) the fluid viscosity, showing the comparison between the experimental data and the theoretical prediction given by equation (1). In the former the fluid viscosity is held constant at 100 mPa.s, and in the latter U =0.185 m s −1 . The SAW frequency is fixed at 19.5 MHz in the latter case. In all cases, error bars denote the s.e. for n =3 runs for each data set. Full size image Fingering instability The images in Figs 1d and 3 show the transverse fingering instability that subsequently develops along the advancing film front. Laser Doppler vibrometer (LDV) scans of the substrate displacement velocity directly beneath the fingers in Fig. 3a reveal the existence of transverse variations in the SAW amplitude. Agreement between the LDV measurements with predictions based upon a Fresnel integral diffraction model (see Supplementary Information for further details of the model), as seen in Fig. 3a , then suggests that the transverse SAW amplitude variation arises as a consequence of Fresnel diffraction due to the finite aperture of the interdigital transducer (IDT) electrode; a modest quantitative discrepancy is present, common in the modelling of Fresnel diffraction phenomena. Given the dependence of the wetting speed of the advancing film front on the SAW amplitude U , apparent from equation (1), such transverse variations in U impose a corresponding fluctuation in the wetting speed across the leading edge of the film and drives a transverse instability that results in the fingering patterns observed in Figs 1d and 3a . 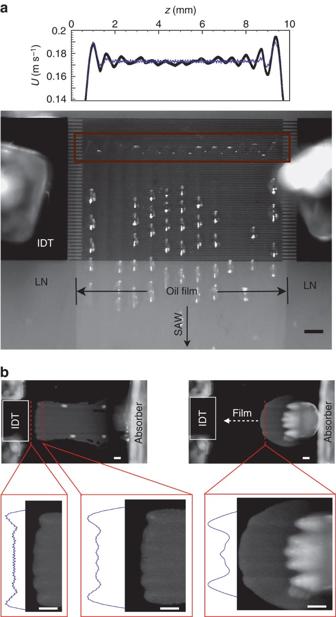Figure 3:Fingering instability. (a) Magnified image of the advancing film front showing the fingering instability triggered by transverse Fresnel diffraction of the underlying SAW directly above the IDT, as measured via an LDV scan of the substrate displacement beneath the fingers (see bold line in the inset above the image). Also shown by the thin blue line in the inset is the displacement predicted by the Fresnel diffraction model, which agrees well with the LDV results. The LDV data is provided as the root-mean square displacement velocity amplitudeUalong the transversez-direction. The scale bar denotes a length of≈1 mm. (b) Similar images of the fingering patterns at positionsλSAW, 10λSAWand 35λSAW(left to right) from the edge of the IDT, respectively, along the SAW propagation axis;λSAWis the SAW wavelength and the scale bars denote lengths of ≈1 mm. A magnified image of the finger patterns for each location is shown below, together with the corresponding transverse displacement velocity amplitudeUpredicted by the Fresnel diffraction model, again showing good qualitative agreement. LN, lithium niobate. Figure 3: Fingering instability. ( a ) Magnified image of the advancing film front showing the fingering instability triggered by transverse Fresnel diffraction of the underlying SAW directly above the IDT, as measured via an LDV scan of the substrate displacement beneath the fingers (see bold line in the inset above the image). Also shown by the thin blue line in the inset is the displacement predicted by the Fresnel diffraction model, which agrees well with the LDV results. The LDV data is provided as the root-mean square displacement velocity amplitude U along the transverse z -direction. The scale bar denotes a length of≈1 mm. ( b ) Similar images of the fingering patterns at positions λ SAW , 10 λ SAW and 35 λ SAW (left to right) from the edge of the IDT, respectively, along the SAW propagation axis; λ SAW is the SAW wavelength and the scale bars denote lengths of ≈1 mm. A magnified image of the finger patterns for each location is shown below, together with the corresponding transverse displacement velocity amplitude U predicted by the Fresnel diffraction model, again showing good qualitative agreement. LN, lithium niobate. Full size image This is further corroborated by favourable comparisons between the fingering patterns and the Fresnel diffraction distribution at progressively longer distances from the IDT along the SAW propagation direction ( Fig. 3b ). The coarser appearance of the fingering fascinatingly corresponds to the broader, longer wavelength features of the Fresnel diffraction, the further away the comparison is made from the IDT that generates the SAW. Curiously, and in further support of Fresnel diffraction as the mechanism responsible for driving the fingering instability, the finger spacing was found to be linearly dependent on the wavelength of the SAW, yet insensitive to changes in the SAW aperture and the ‘gap’ between the individual IDT finger tips and the adjacent bus bar ( Fig. 4 ). 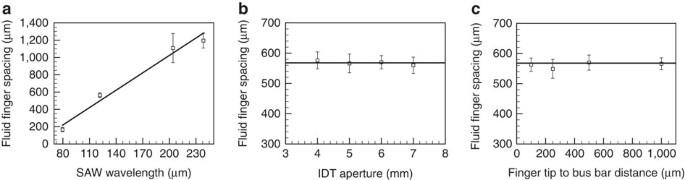Figure 4:Effect of various system parameters on the characteristic finger spacing. Dependence of the characteristic spacing of the fingering patterns on (a) the SAW wavelength (and hence frequency), (b) the IDT aperture, and (c) the ‘gap’ between the IDT finger tip and bus bar. The measurement is made when the advancing front of the film, where the finger patterns develop, reaches the middle of the IDT. When not varied, the SAW frequency, IDT aperture and distance between the IDT finger tip and bus bar are held constant at 32.7 MHz, 7 mm and 500 μm, respectively. It can be seen that the fluid finger spacing is almost linearly dependent (R2=0.98) on the SAW wavelength, but is independent of the IDT design. The error bars denote the s.e. forn=10 finger patterns for each point. Figure 4: Effect of various system parameters on the characteristic finger spacing. Dependence of the characteristic spacing of the fingering patterns on ( a ) the SAW wavelength (and hence frequency), ( b ) the IDT aperture, and ( c ) the ‘gap’ between the IDT finger tip and bus bar. The measurement is made when the advancing front of the film, where the finger patterns develop, reaches the middle of the IDT. When not varied, the SAW frequency, IDT aperture and distance between the IDT finger tip and bus bar are held constant at 32.7 MHz, 7 mm and 500 μm, respectively. It can be seen that the fluid finger spacing is almost linearly dependent ( R 2 =0.98) on the SAW wavelength, but is independent of the IDT design. The error bars denote the s.e. for n =10 finger patterns for each point. Full size image Wave generation and propagation The finger formation is followed by the emergence of wave pulses (see Figs 1d , e and ), which, from Fig. 5 , appear to grow mainly from the capillary ridges above the advancing film front and eventually translate away in the direction reverse to that of the film spreading (that is, along the SAW propagation direction), exhibiting soliton-like behaviour and maintaining a constant volume. The dimensions of the wave pulses were found to be insensitive to the SAW power and fluid properties, only depending on the wavelength of the SAW. We attribute the initial growth of the film ( Fig. 5a ) to the continued flow into the capillary ridge, as the film spreading is arrested at a specific location along the IDT. 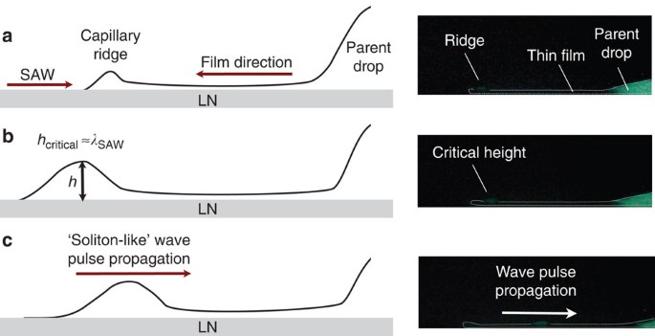Figure 5:Generation and propagation of soliton-like wave pulses. Schematic (left) and fluorescent images (right) showing (a) the capillary ridge at the leading edge of the advancing film front pulled out from the parent drop in the direction opposing that of the SAW propagation. (b) The capillary ridge subsequently grows when the film is prohibited from spreading further to form (c) a ‘soliton-like’ wave pulse that propagates away in the direction opposite to that of the film spreading once the film heighthreaches a threshold valuehcritical≈λSAWat which point Eckart streaming begins to dominate;λSAWbeing the SAW wavelength. Dashed lines were added to aid visualisation of the thin film. LN, lithium niobate. Figure 5: Generation and propagation of soliton-like wave pulses. Schematic (left) and fluorescent images (right) showing ( a ) the capillary ridge at the leading edge of the advancing film front pulled out from the parent drop in the direction opposing that of the SAW propagation. ( b ) The capillary ridge subsequently grows when the film is prohibited from spreading further to form ( c ) a ‘soliton-like’ wave pulse that propagates away in the direction opposite to that of the film spreading once the film height h reaches a threshold value h critical ≈ λ SAW at which point Eckart streaming begins to dominate; λ SAW being the SAW wavelength. Dashed lines were added to aid visualisation of the thin film. LN, lithium niobate. Full size image More specifically, the growth of the capillary ridge to form a solitary wave-like structure can be attributed to continued inflow into the nose of the film due to Rayleigh streaming, as long as the film front is prohibited from further spreading and as long as there is no mechanism for outflow away from the ridge region. The former occurs because the SAW is partially composed of a standing wave within the IDT and assumes a complete standing wave form at some location along the IDT. The latter is true as long as the height of the film and ridge remain sufficiently small, such that the confinement provided by their thicknesses prohibit sufficient pathlength to attenuate the energy leaked into the fluid by the SAW to drive Eckart streaming. Given that the dominance of Rayleigh streaming over Eckart streaming begins to wane as the ridge (wave pulse) thickness h exceeds λ l , it is reasonable to assume that the ridge (wave pulse) grows to this critical threshold height h critical ≈ λ SAW > λ l before being transported away in the opposing direction due to the now-dominant Eckart flow. This is verified by experimental measurements of h critical , which appear to strongly correspond to λ SAW irrespective of the viscosity, frequency or input voltage (see Fig. 6 , inset). 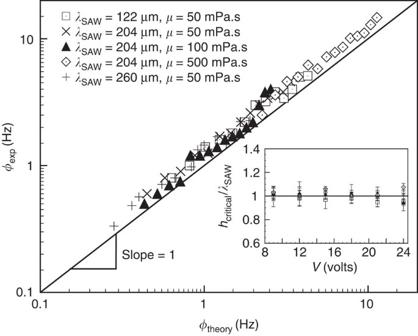Figure 6:Wave pulse generation rate. Comparison between the frequency Φ at which the wave pulses are generated, predicted by applying volume conservation across a control volume around the capillary ridge region, with experimentally measured data. The inset shows the critical heighthcritical(normalised by the SAW wavelengthλSAW) to which the capillary ridge (wave pulse) grows before it translates away under Eckart flow. This is measured as a function of the applied power for different frequencies and liquid viscosities. The error bars are the s.e. forn=5 wave pulse size measurements for each point. Figure 6: Wave pulse generation rate. Comparison between the frequency Φ at which the wave pulses are generated, predicted by applying volume conservation across a control volume around the capillary ridge region, with experimentally measured data. The inset shows the critical height h critical (normalised by the SAW wavelength λ SAW ) to which the capillary ridge (wave pulse) grows before it translates away under Eckart flow. This is measured as a function of the applied power for different frequencies and liquid viscosities. The error bars are the s.e. for n =5 wave pulse size measurements for each point. Full size image Volume conservation applied over a control volume around the capillary ridge region then permits an estimation of the rate at which these wave pulses appear, as the rate at which each capillary ridge (wave pulse) height grows must equal the volumetric inflow rate into the capillary ridge region. Given that the latter can be estimated from the velocity (equation (1)) and film thickness (≈20 μm), the rate at which these wave pulses are generated can then be predicted if it is assumed that the capillary ridge grows to h critical before translating away. The close agreement in Fig. 6 not only verifies the postulated reason for the existence and transport of the wave pulses but also supports the proposed mechanism underpinning the spreading dynamics, which form the basis on which equation (1) is derived. In summary, we report and elucidate for the first time the rich dynamics associated with three combined phenomena, all originating from a single sessile drop when it is subjected to nanoscale-amplitude, substrate wave vibrations in the form of SAWs: film spreading, fingering instabilities and ‘soliton-like’ wave propagation. The spreading of the film, drawn out from the sessile drop, opposes the direction of the SAW propagation and is a consequence of Rayleigh-streaming-driven drift flow, whereas the subsequent instability of the advancing film front to produce fingering patterns is triggered by perturbations imposed on the front due to transverse Fresnel diffraction of the underlying acoustic wave. Above the fingers, discrete wave packets are then observed to form and translate in the direction of the SAW propagation away from the leading edge of the film, which we attribute to reversal of the flow as a consequence of the transition from Rayleigh streaming, dominant in the thin film, to Eckart streaming, dominant when the fluid (that is, the wave packet) reaches a critical thickness corresponding to the SAW wavelength. Apart from uncovering further peculiarities associated with wetting phenomena that has a rich and storied history dating back to Thomson’s [31] discovery (and Marangoni’s [32] subsequent analysis) of ‘wine tears’ and the complex physico-chemical hydrodynamics that accompany such phenomena, we anticipate the ability to finely control the spreading of fluids using acoustic fields will drive further technological advances in film coating (especially thick photoresist coating) and microfluidic transport (as a microdroplet generator, for example, upon ejection of the wave packets from the substrate edge) for diverse applications from point-of-care diagnostics and drug screening to biosensing and drug delivery [13] . Device The experimental setup, schematically depicted in Fig. 1a , comprised a 10-nm chrome/250-nm aluminium IDT electrode photolithographically patterned on a 0.5-mm thick 128 o Y -cut, X -propagating single-crystal lithium niobate piezoelectric substrate. Forty-two electrode finger pairs were used, with a distance of 100, 250, 500 or 1,000 μm between the tips of the IDT fingers and the bus bar. Different IDT apertures (4, 5, 6 and 7 mm) were fabricated and tested; each configuration was designed to operate at either 50, 32.7, 19.5 or 15.3 MHz. An absorbent (α-gel, Geltec Ltd, Yokohama, Japan) was placed along the edge of the device to eliminate wave reflections. Surface acoustic wave The SAW, a nanometer-order amplitude Rayleigh wave, is generated by applying a sinusoidal electric field to the IDT at resonance using a signal generator (SML01, Rhode & Schwarz, North Ryde, NSW, Australia) and amplifier (10W1000C, Amplifier Research, Souderton, PA, USA), the SAW wavelength λ SAW (and hence the frequency f ) being determined by the width and gap of the IDT finger patterns. The actual voltage across the device was measured using an oscilloscope (Wavejet 332/334, LeCroy, Chestnut Ridge, NY, USA), and spatiotemporal variations in the wave displacement and velocity amplitude along the underlying substrate were measured using a LDV (UHF-120, Polytec GmBH, Waldbronn, Germany). Materials Silicone oil (Sigma-Aldrich Pty Ltd, North Ryde, NSW, Australia) as the working fluid with viscosity μ ≈50, 100 and 500 mPa.s and density ρ ≈1,000 kg m −3 was dyed using trace quantities of fluorescent dye (Dye-Lite TP-3400-0601, Tracer Products, Westbury, NY, USA) to enhance visualisation, captured using a digital SLR camera (EOS 550D, Canon, Utsnomiya, Japan) fitted with a macro lens (EF-S, Canon; 60 mm focal length, F/2.8). To render the substrate oleophobic to silicone oil, we patterned a 100-nm thick Teflon (Teflon AF, DuPont Corp., Wilmington, DE, USA) layer onto the substrate. How to cite this article: Rezk, A. R. et al. Unique fingering instabilities and soliton-like wave propagation in thin acoustowetting films. Nat. Commun. 3:1167 doi: 10.1038/ncomms2168 (2012).